UTX coordinates steroid hormone-mediated autophagy and cell death Correct spatial and temporal induction of numerous cell type-specific genes during development requires regulated removal of the repressive histone H3 lysine 27 trimethylation (H3K27me3) modification. Here we show that the H3K27me3 demethylase dUTX is required for hormone-mediated transcriptional regulation of apoptosis and autophagy genes during ecdysone-regulated programmed cell death of Drosophila salivary glands. We demonstrate that dUTX binds to the nuclear hormone receptor complex Ecdysone Receptor/Ultraspiracle, and is recruited to the promoters of key apoptosis and autophagy genes. Salivary gland cell death is delayed in dUTX mutants, with reduced caspase activity and autophagy that coincides with decreased apoptosis and autophagy gene transcripts. We further show that salivary gland degradation requires dUTX catalytic activity. Our findings provide evidence for an unanticipated role for UTX demethylase activity in regulating hormone-dependent cell death and demonstrate how a single transcriptional regulator can modulate a specific complex functional outcome during animal development. Programmed cell death (PCD) is essential for animal development and is required for tissue modelling, deleting harmful cells and to maintain homeostasis. In response to various signals such as cytotoxic insults, hormones and growth factors the control of the transcriptional balance between pro-survival and pro-death genes can modulate PCD. Nuclear hormone receptors (NR) play essential roles in spatial and temporal regulation of gene transcription as they recruit histone-modifying enzymes to gene promoters/enhancers [1] , [2] . These multi-protein complexes modulate the expression of distinct gene networks regulating diverse biological processes such as cell proliferation, differentiation and PCD [1] , [2] , [3] . An important determinant of the transcriptional status of a gene is the histone methylation profile. The methylation of lysine residues on histones is site-specific and highly regulated by histone lysine methyltransferases (KMT) and lysine demethylases (KDM) [4] , [5] . Generally, methylation of histone 3 on lysine 4 (H3K4), lysine 36 (H3K36) and lysine 79 (H3K79) is associated with active transcription, whereas methylation of lysine 9 (H3K9) and lysine 27 (H3K27) is associated with repression. Depending on the context, histone methylation patterns may be stably maintained or amenable to change. The highly conserved Polycomb group (PcG) and Trithorax group (TrxG) complexes are critical regulators of numerous developmental genes that act antagonistically in the maintenance of transcriptional repression or activation, respectively [6] . The PcG protein EZH2 is a KMT that trimethylates H3K27 facilitating gene repression. For gene expression, H3K27me3 is removed and promoters acquire H3K4me3 mediated by TrxG complexes [7] , [8] . The Jumonji (JMJ) domain-containing histone demethylases (HDMs) JMJD3 and UTX antagonize PcG-mediated silencing by removing the repressive methylation mark from H3K27me3, leading to an active chromatin state [9] , [10] , [11] , [12] , [13] , [14] . Recent studies have uncovered several roles for UTX including differentiation of mesoderm, embryonic stem cells and haematopoietic cells, cardiac development and myogenesis by remodelling chromatin, and facilitating the recruitment of appropriate transcriptional factors [15] , [16] , [17] , [18] . In addition to the demethylase functions, UTX appears to have enzyme-independent functions. While Utx is essential for murine embryonic viability and development, this is independent of demethylase function as Uty, which lacks demethylase activity, is able to compensate for Utx [19] , [20] , [21] . In addition, UTX associates with TrxG KMT (MLL2/3/4) and has demethylase-independent functions [22] , [23] . However, the roles of UTX in these demethylase-independent functions remain controversial. The association of UTX with MLL and the importance of MLL complexes in NR-mediated gene regulation suggest that UTX may play a role in hormone-dependent transcriptional control. Indeed, several KDMs act as coregulators with the androgen receptor; however, a role for UTX in androgen receptor-mediated transcription has not yet been identified [8] . Despite the growing evidence for the role of H3K27 methylation in transcriptional regulation in stem cells, cell proliferation and cancer, the understanding of its role in hormone-dependent transcription and PCD is limited. Nuclear receptor signaling pathways are highly conserved and in Drosophila the steroid hormone, 20-hydroxyecdysone (ecdysone), forms a complex with its heterodimeric nuclear hormone receptor, Ecdysone Receptor/Ultraspiracle (EcR/Usp), to modulate the transcription of many genes during major developmental transitions [1] , [24] . Following the larval–pupal transition a rise in ecdysone triggers the PCD of larval tissues no longer needed including the salivary glands [25] . The removal of the salivary glands depends on both apoptosis and autophagy and when both pathways are inhibited salivary gland PCD is blocked [26] . The expression of both apoptosis and autophagy genes is increased in dying salivary glands [26] , [27] , [28] , [29] , [30] . The transcriptional upregulation of the apoptosis initiator reaper ( rpr ), caspase genes dronc and drice , and the adaptor dark in response to ecdysone is in part due to the direct binding of EcR/Usp to these promoters recruiting histone-modifying enzymes to activate apoptotic genes in specific tissues [31] , [32] , [33] , [34] , [35] , [36] . Here we show that the Drosophila H3K27 demethylase orthologue, dUTX, drives temporal regulation of apoptosis and autophagy genes during ecdysone-mediated PCD of the salivary glands. Our data suggest that a physical association between dUTX and EcR/Usp results in their recruitment to promoters of key cell death and autophagy genes leading to H3K27me3 demethylation and subsequent gene expression during ecdysone-mediated PCD. dUTX interacts with EcR and regulates ecdysone-induced PCD Active gene transcription is generally associated with H3K4 trimethylation and removal of H3K9 and H3K27 trimethylation. We have found that in response to the hormone ecdysone, H3 associated with the promoters of cell death genes dronc , which encodes the essential apoptotic caspase in Drosophila and dark , which encodes the adaptor protein required for Dronc activation, acquires H3K4me3 while losing H3K9me3 (ref. 36 ). This suggests that HDMs are recruited to the promoters of key cell death genes to remove repressive histone marks such as H3K9me3 and H3K27me3 during hormone-mediated transcription. To determine which of the Jumonji HDM family members in Drosophila regulate PCD, we undertook a cell-based RNAi screen using cell lines that undergo ecdysone-mediated cell death [37] . Among the genes tested, we found that dUTX knockdown resulted in significantly reduced ecdysone-mediated cell death and caspase activity ( Fig. 1 ). As dUTX encodes a H3K27me3 demethylase, this suggested that the removal of H3K27me3 may be important in hormone-mediated transcriptional control of PCD. 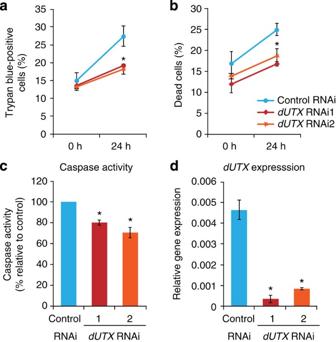Figure 1: dUTX regulates ecdysone-induced cell death. (a–d) RNAi-mediated knockdown ofdUTXinhibits ecdysone-induced apoptotic cell death. SL2 cells were treated with two independent dsRNAs todUTXor a control gene (GFP) for 48 h and cell death was induced with 10 μM ecdysone for 24 h. (a) The cell viability was assayed by trypan blue staining. Data are mean from three independent experiments, with error bars representing s.e.m. *P<0.05 (Student’st-test). (b) Cell count and viability assay using Muse (Millipore, USA). Data are mean from three independent experiments, with error bars representing s.d. *P<0.05 (Student’st-test). (c) Caspase activity was measured from total cell lysate on DEVD-AMC, represented as fold increase relative to control RNAi. Data are mean from three independent experiments, with error bars representing s.e.m. *P<0.05 (Student’st-test). (d) The level of knockdown ofdUTXwas quantificated by qPCR and normalized against ribosomal proteinrp49. Relative dUTX expression levels following knockdown using the two independent dsRNA are shown (n=3) with error bars representing s.d. *P<0.05 (Student’st-test). Figure 1: dUTX regulates ecdysone-induced cell death. ( a – d ) RNAi-mediated knockdown of dUTX inhibits ecdysone-induced apoptotic cell death. SL2 cells were treated with two independent dsRNAs to dUTX or a control gene (GFP) for 48 h and cell death was induced with 10 μM ecdysone for 24 h. ( a ) The cell viability was assayed by trypan blue staining. Data are mean from three independent experiments, with error bars representing s.e.m. * P <0.05 (Student’s t -test). ( b ) Cell count and viability assay using Muse (Millipore, USA). Data are mean from three independent experiments, with error bars representing s.d. * P <0.05 (Student’s t -test). ( c ) Caspase activity was measured from total cell lysate on DEVD-AMC, represented as fold increase relative to control RNAi. Data are mean from three independent experiments, with error bars representing s.e.m. * P <0.05 (Student’s t -test). ( d ) The level of knockdown of dUTX was quantificated by qPCR and normalized against ribosomal protein rp49 . Relative dUTX expression levels following knockdown using the two independent dsRNA are shown ( n =3) with error bars representing s.d. * P <0.05 (Student’s t -test). Full size image The temporal expression of the key apoptotic caspases dronc and drice during hormone-mediated PCD requires the binding of EcR/Usp directly to their promoter to enable the recruitment of coactivators [33] , [34] , [35] , [38] . Nuclear receptor coactivators frequently contain a LXXLL or LLXXL nuclear-receptor-interacting motif and sequence analysis of dUTX identified a potential motif LLQTL (amino acids 1,033–1,037 in isoform dUTX-RA) in the C-terminal region, which is conserved in mammalian UTX (LLRTL) [39] . To determine whether the role of dUTX in cell death was through an interaction with EcR/Usp, we examined the interaction between the C-terminal region of dUTX containing the LLQTL motif (dUTX–NR) and in vitro translated 35 S-labelled EcR/Usp. A direct association between dUTX–NR and EcR/Usp was observed both in the presence and absence of ecdysone ( Fig. 2a ). This interaction was confirmed in cells where endogenous EcR immunoprecipitated with HA-dUTX both in the presence and absence of ecdysone ( Fig. 2b ). In addition, colocalization of EcR and dUTX was observed in vivo on salivary gland polytene chromosomes ( Fig. 2c ). 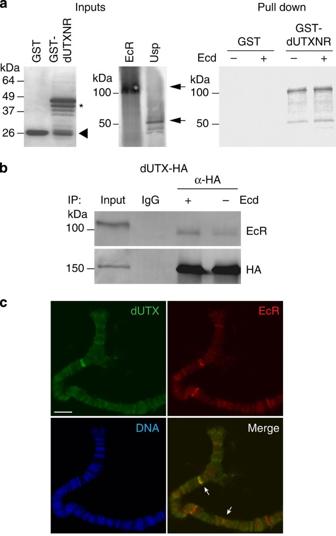Figure 2: dUTX directly interacts with ecdysone receptor. (a,b) dUTX directly interacts with ecdysone receptor (EcR/Usp). (a) GST and GST-dUTX–NR containing the nuclear hormone domain were used in pull-down experiments with35S-labelled EcR and Usp in the presence of ethanol control (−) or 10 μM ecdysone (+). The GST input proteins are shown in Coomassie Brilliant blue-stained gel, GST is labelled with arrow head and dUTX–NR with an asterisk. The EcR and Usp inputs are shown labelled with arrows. (b) Immunoprecipitation (IP) of EcR and dUTX in SL2 cells. Cells were transfected with HA-dUTX and the cell lysates were immunoprecipitated using anti-HA or a control IgG isotype antibody. The immunoprecipitates were analysed by western blotting using the anti-EcR and anti-HA antibodies. (c) Colocalization of dUTX and EcR on salivary gland polytene chromosomes. Immunostaining of salivary glands polytene chromosome prepared from third instar larvae expressing FLAG-dUTX with dUTX (green) and EcR (red), with Hoechst-stained DNA (blue). Arrows indicate examples of colocalized bands. No signal was detected when immunostaining with secondary antibody only. Scale bar represent 5 μm. Figure 2: dUTX directly interacts with ecdysone receptor. ( a , b ) dUTX directly interacts with ecdysone receptor (EcR/Usp). ( a ) GST and GST-dUTX–NR containing the nuclear hormone domain were used in pull-down experiments with 35 S-labelled EcR and Usp in the presence of ethanol control (−) or 10 μM ecdysone (+). The GST input proteins are shown in Coomassie Brilliant blue-stained gel, GST is labelled with arrow head and dUTX–NR with an asterisk. The EcR and Usp inputs are shown labelled with arrows. ( b ) Immunoprecipitation (IP) of EcR and dUTX in SL2 cells. Cells were transfected with HA-dUTX and the cell lysates were immunoprecipitated using anti-HA or a control IgG isotype antibody. The immunoprecipitates were analysed by western blotting using the anti-EcR and anti-HA antibodies. ( c ) Colocalization of dUTX and EcR on salivary gland polytene chromosomes. Immunostaining of salivary glands polytene chromosome prepared from third instar larvae expressing FLAG-dUTX with dUTX (green) and EcR (red), with Hoechst-stained DNA (blue). Arrows indicate examples of colocalized bands. No signal was detected when immunostaining with secondary antibody only. Scale bar represent 5 μm. Full size image dUTX is required for larval salivary gland cell death During metamorphosis the removal of obsolete larval salivary glands occurs in response to a developmental pulse of ecdysone 10–12 h relative to puparium formation (RPF). To investigate the role of dUTX in ecdysone-mediated PCD in vivo , we examined the removal of the salivary glands in the loss-of-function dUTX mutant, dUTX 1 . dUTX is essential for development, with dUTX deficiency resulting in pupal lethality, with a small percentage of escapers that die immediately following eclosion [23] . In control animals the salivary glands were intact at 12 h RPF and were degraded with only small tissue fragments remaining by 24 h RPF ( Fig. 3a ). In contrast, the degradation of the dUTX 1 salivary glands was significantly delayed, as intact salivary glands were present in many animals at 24 h RPF ( Fig. 3a ). A similar phenotype was also observed in a heteroallelic combination of dUTX mutants ( Supplementary Fig. S1 ). These results indicate that dUTX is required for the ecdysone-mediated PCD of larval salivary glands during metamorphosis. 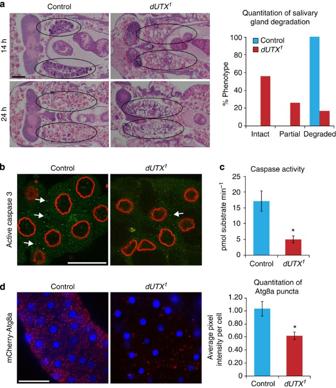Figure 3: dUTX is required for salivary gland cell death. (a) Histological analysis of paraffin sections at 14 h and 24 h RPF shows intact salivary glands present indUTX1compared with control at 24 h RPF. Ovals indicate the position of salivary glands and fragments. Scale bar represent 50 μm. Quantification of the salivary gland phenotypic data was at 24 h RPF. (b,c) Caspase staining and activity are reduced indUTX1salivary glands at 14 h RPF. (b) Cleaved caspase-3 antibody (green) and Lamin antibody (red) staining are shown in control anddUTX1salivary glands at 14 h RPF. Scale bar represents 50 μm. (c) Caspase activity was measured from 14 h RPF control anddUTX1salivary glands using DEVD-AMC as a substrate. Data are mean from three independent experiments each using at least 20 salivary glands from control anddUTX1for preparing cell extracts. The error bars represent s.e.m. *P-value<0.05 (Student’st-test). (d) Autophagy puncta examined using mCherry-Atg8a (red) and nuclei stained with Hoechst (blue). Scale bar represents 100 μm. The quantitation of the mCherry-Atg8a puncta as the mean fluorescent pixel intensity per cell (controln=242,dUTX1n=224), with error bars representing s.e.m. *P-value<0.05 (Student’st-test). Figure 3: dUTX is required for salivary gland cell death. ( a ) Histological analysis of paraffin sections at 14 h and 24 h RPF shows intact salivary glands present in dUTX 1 compared with control at 24 h RPF. Ovals indicate the position of salivary glands and fragments. Scale bar represent 50 μm. Quantification of the salivary gland phenotypic data was at 24 h RPF. ( b , c ) Caspase staining and activity are reduced in dUTX 1 salivary glands at 14 h RPF. ( b ) Cleaved caspase-3 antibody (green) and Lamin antibody (red) staining are shown in control and dUTX 1 salivary glands at 14 h RPF. Scale bar represents 50 μm. ( c ) Caspase activity was measured from 14 h RPF control and dUTX 1 salivary glands using DEVD-AMC as a substrate. Data are mean from three independent experiments each using at least 20 salivary glands from control and dUTX 1 for preparing cell extracts. The error bars represent s.e.m. * P -value<0.05 (Student’s t -test). ( d ) Autophagy puncta examined using mCherry-Atg8a (red) and nuclei stained with Hoechst (blue). Scale bar represents 100 μm. The quantitation of the mCherry-Atg8a puncta as the mean fluorescent pixel intensity per cell (control n =242, dUTX 1 n =224), with error bars representing s.e.m. * P -value<0.05 (Student’s t -test). Full size image To investigate the in vivo interaction between dUTX and EcR we examined the RNAi-mediated knockdown of EcR in the salivary glands of dUTX 1 animals. As EcR has an essential function in salivary gland removal knockdown of EcR in the salivary glands results in the persistence of salivary glands well beyond the normal timing of their PCD in the controls ( Supplementary Fig. S2 ). This strong salivary gland phenotype associated with EcR knockdown was not suitable for dose-dependent genetic modification. However, we were able to examine the timing of the lethality of dUTX 1 animals where EcR levels were reduced by RNAi. Homozygous dUTX 1 animals survive past the morphological process of head eversion (12 h RPF) and die before eclosion. When EcR was knocked down in a dUTX 1 mutant background, the proportion of animals that survived to head eversion was significantly reduced compared with dUTX 1 alone ( Table 1 ). This result, showing that depletion of EcR in the salivary glands of dUTX 1 enhances the lethality, implies an in vivo genetic interaction between dUTX and EcR. Table 1 Combined loss of dUTX and EcR increases lethality of dUTX Full size table dUTX regulates apoptosis and autophagy in salivary glands A critical step required for salivary gland PCD is the induction of apoptosis, resulting in the activation of initiator caspase Dronc and effector caspase Drice [27] , [28] . We examined whether the delayed degradation of the salivary glands observed in dUTX 1 was due to reduced caspase activity. Salivary glands were stained with an antibody to cleaved caspase-3 (that represents active caspases) at 14 h RPF and compared with controls, the dUTX 1 salivary glands showed reduced immunostaining ( Fig. 3b ; Supplementary Fig. S3 ). Consistent with this, bulk caspase activity as determined by substrate cleavage, at 14 h RPF was significantly lower in dUTX 1 salivary glands compared with the control ( Fig. 3c ). The complete removal of the larval salivary glands requires both apoptosis as well as autophagy, and blocking either pathway alone results in delayed degradation [26] . To determine whether the delayed removal of salivary glands in dUTX 1 was also due to reduced autophagy we examined the levels of mCherry–Atg8a puncta formation [40] . In the control salivary glands, high levels of puncta were clearly evident at 14 h RPF; however, dUTX 1 salivary glands showed reduced puncta at the same time ( Fig. 3d ). This suggests that in addition to impaired caspase activity there is also a reduction in autophagy, coinciding with delayed removal of the salivary glands in dUTX mutant animals. As removal of the salivary glands is triggered by ecdysone, the defects observed in the dUTX mutant animals could potentially be due to a more general defect in ecdysone synthesis and levels. If dUTX has a role in the production of ecdysone, it is likely to be at the level of transcription of ecdysone biosynthesis genes. We examined the expression of genes involved in ecdysone biosynthesis and found that their transcript levels in dUTX 1 animals were comparable to the transcript levels in the control animals at the same stage ( Supplementary Fig. S4a ). Additionally, the levels of ecdysone assessed at 12 h RPF were unaffected in the dUTX 1 animals ( Supplementary Fig. S4b ), suggesting that dUTX does not affect ecdysone production or levels. These findings are consistent with the observations that dUTX 1 animals undergo morphological changes during metamorphosis, including pupariation (0 h RPF) and head eversion (12 h RPF), indicating that other ecdysone-regulated processes are not affected. As stated above, the majority of dUTX 1 animals fail to progress through later developmental stages and die [23] . dUTX regulates expression of apoptosis and autophagy genes As an H3K27me3 demethylase, dUTX may be recruited by EcR/Usp to the promoters of specific genes to remove the repressive epigenetic mark. Given the reduction in caspase activity observed in dUTX mutant salivary glands, we investigated whether the expression of apoptosis genes was altered in the absence of dUTX . Previous studies have shown that ecdysone regulates transcription of dronc , drice , dark and rpr to induce salivary gland PCD [31] , [32] , [33] , [34] , [35] , [36] . An examination of the transcriptional profile of dronc , drice , dark and rpr showed similar transcript levels for these genes in control and dUTX 1 salivary glands prior to cell death at 6 h RPF ( Fig. 4a ). Following initiation of cell death at 14 h RPF, dronc , drice and rpr expression was induced in the control salivary glands; however in the dUTX 1 salivary glands there were significantly lower transcript levels of these genes ( Fig. 4a ). 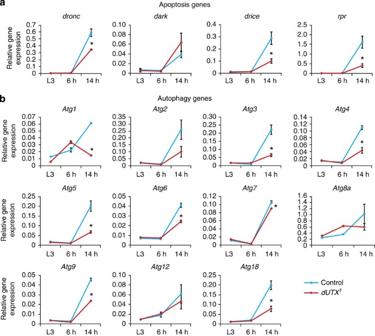Figure 4:dUTX regulates ecdysone-mediated transcription of PCD andAtggenes. (a) Levels ofdark,dronc,driceandrprtranscripts were measured from third instar larvae (L3), 6 h and 14 h RPF salivary glands from control (blue) anddUTX1(red) by qPCR and expressed relative to the internal control generp49. (b) The transcript levels ofAtggenes relative to the internal control generp49in the salivary glands of control (blue) anddUTX1(red) were analysed by qPCR at L3, 6 h and 14 h RPF. Data in all panels are expressed as means from three independent experiments, with error bars representing s.e.m. *P<0.05 (Student’st-test). Figure 4: dUTX regulates ecdysone-mediated transcription of PCD and Atg genes. ( a ) Levels of dark , dronc , drice and rpr transcripts were measured from third instar larvae (L3), 6 h and 14 h RPF salivary glands from control (blue) and dUTX 1 (red) by qPCR and expressed relative to the internal control gene rp49 . ( b ) The transcript levels of Atg genes relative to the internal control gene rp49 in the salivary glands of control (blue) and dUTX 1 (red) were analysed by qPCR at L3, 6 h and 14 h RPF. Data in all panels are expressed as means from three independent experiments, with error bars representing s.e.m. * P <0.05 (Student’s t -test). Full size image As there was also a reduction in autophagy levels in the dUTX 1 salivary glands, we investigated whether the expression of autophagy genes were altered in the absence of dUTX . The transcript levels of several Autophagy-related ( Atg ) genes have been shown to increase in salivary glands at 14 h RPF [29] , [30] . Prior to the induction of PCD at 6 h RPF the transcript levels of the Atg genes examined remained at low levels in dUTX 1 similar to the control ( Fig. 4b ). However, at 14 h RPF there was significantly reduced expression of several Atg genes, including Atg1 , Atg3 , Atg4 , Atg5 , Atg6 , Atg7 , Atg9 and Atg18 , in dUTX 1 compared with control where the expression of Atg genes was higher ( Fig. 4b ). The lower levels of apoptosis and autophagy gene transcripts in dUTX 1 salivary gland at the time of PCD suggests that dUTX plays an important role in maintaining the correct temporal regulation of the transcriptional response to ecdysone. dUTX is recruited to apoptosis and autophagy gene promoters The findings above imply that dUTX is recruited to cell death gene promoters to control the timing of the hormone-mediated removal of the salivary glands. To examine the recruitment of dUTX to the promoters of the ecdysone-responsive genes, we performed chromatin immunoprecipitation (ChIP) assays using SL2 cells transfected with tagged dUTX following treatment with ecdysone. dUTX was recruited to the promoter of apoptosis genes dark , dronc , drice and rpr ( Fig. 5a ). Furthermore, we observed recruitment of dUTX on several Atg gene promoters, including Atg1 , Atg2 , Atg3 , Atg4 , Atg5 , Atg6 , Atg7 , Atg8a , Atg9 and Atg18 , but not on the Atg12 promoter ( Fig. 5b ). This is consistent with the expression profile of these genes during salivary gland cell death, where dUTX 1 did not show significantly different levels of Atg12 transcripts. The demethylase activity of dUTX targets H3K27me3 so we would predict that in the absence of dUTX the promoters of the apoptosis and autophagy genes would maintain higher levels of H3K27me3. In dUTX knockdown cells ChIP analysis using H3K27me3 shows enrichment of H3K27me3 on the promoters of several apoptosis and autophagy genes ( Fig. 5c ). The promoters of apoptosis genes dark and rpr as well as autophagy genes, Atg1 , Atg2 , Atg7 , Atg9 and Atg18 showed significantly increased H3K27me3. The minor discrepancies detected between dUTX knockdown cells and dUTX 1 animals most likely reflect the molecular differences between ecdysone-induced cell death in the cell line compared with that in vivo . 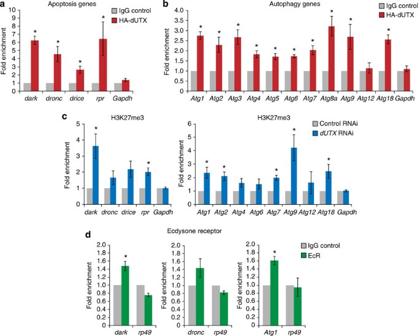Figure 5:dUTX is recruited to the promoters of apoptosis andAtggenes. (a,b) The occupancy of dUTX on the promoter regions of apoptosis andAtggenes was detected by chromatin immunoprecipitation (ChIP). SL2 cells overexpressing HA-dUTX were chromatin-immunoprecipitated with anti-HA and anti-GFP (IgG control) antibodies following ecdysone treatment. qPCR was used to assess the binding to the promoters ofdark,dronc,driceandrpr(a) andAtg1,Atg2,Atg3,Atg4,Atg5,Atg6,Atg7,Atg8a,Atg9,Atg12andAtg18(b), expressed relative to the internal control geneGapdh.Results are shown as the fold enrichment of % input compared with IgG control. (c) The abundance of H3K27me3 on the promoters of apoptosis and autophagy genes detected by ChIP. SL2 cells knocked down fordUTXwere chromatin-immunoprecipitated with anti-H3K27me3 and anti-GFP (IgG control) antibodies following ecdysone treatment. Results are shown as the fold enrichment of % input compared with RNAi control. (d) The occupancy of EcR on the promoter regions ofdark,droncandAtg1by ChIP expressed relative to the internal control generp49. Chromatin was immunoprecipitated with anti-EcR-B1 and anti-GFP (IgG control) antibodies from SL2 cell following ecdysone treatment. Results are shown as the fold enrichment of % input compared with IgG control. Data in all panels are expressed as means from three independent experiments, with error bars representing s.e.m. *P<0.05 (Student’st-test). Figure 5: dUTX is recruited to the promoters of apoptosis and Atg genes. ( a , b ) The occupancy of dUTX on the promoter regions of apoptosis and Atg genes was detected by chromatin immunoprecipitation (ChIP). SL2 cells overexpressing HA-dUTX were chromatin-immunoprecipitated with anti-HA and anti-GFP (IgG control) antibodies following ecdysone treatment. qPCR was used to assess the binding to the promoters of dark , dronc , drice and rpr ( a ) and Atg1 , Atg2 , Atg3 , Atg4 , Atg5 , Atg6 , Atg7 , Atg8a , Atg9 , Atg12 and Atg18 ( b ), expressed relative to the internal control gene Gapdh. Results are shown as the fold enrichment of % input compared with IgG control. ( c ) The abundance of H3K27me3 on the promoters of apoptosis and autophagy genes detected by ChIP. SL2 cells knocked down for dUTX were chromatin-immunoprecipitated with anti-H3K27me3 and anti-GFP (IgG control) antibodies following ecdysone treatment. Results are shown as the fold enrichment of % input compared with RNAi control. ( d ) The occupancy of EcR on the promoter regions of dark , dronc and Atg1 by ChIP expressed relative to the internal control gene rp49 . Chromatin was immunoprecipitated with anti-EcR-B1 and anti-GFP (IgG control) antibodies from SL2 cell following ecdysone treatment. Results are shown as the fold enrichment of % input compared with IgG control. Data in all panels are expressed as means from three independent experiments, with error bars representing s.e.m. * P <0.05 (Student’s t -test). Full size image While the expression data show that the transcript levels of Atg genes increase following ecdysone, it is not known if this is due to the direct binding of EcR/Usp to the promoters or secondary transcription factors. As Atg1 is a key upstream regulator of autophagy, we examined the Atg1 promoter sequence for potential EcR consensus DNA-binding sequence and identified a region +335 nucleotides from the transcription start site. Given our findings that dUTX is recruited to the Atg1 gene promoter we predicted that EcR would also be present at this promoter. Consistent with previous studies, following ecdysone treatment, there was an increase in EcR-B1 recruitment on the dronc and dark promoters ( Fig. 5d ). In addition, using primers spanning the potential EcR-binding sequence we also detected the recruitment of EcR-B1 to the Atg1 promoter ( Fig. 5d ). Taken together, these data provide a model whereby EcR/Usp recruits dUTX to the promoters of apoptosis and autophagy genes, required for the temporal induction of transcription in response to ecdysone during salivary gland PCD. This is an important finding, as UTX family members have not previously been implicated in hormone-mediated transcription of apoptosis and autophagy genes. dUTX regulates expression of E93 In addition to the direct regulation of apoptosis gene expression by EcR/Usp, a transcriptional hierarchy is triggered in response to ecdysone whereby EcR/Usp (along with the βFTZ-F1 orphan nuclear receptor) directly activates transcription of the early genes Broad Complex ( BR-C ), E74 and E93 [41] , [42] , [43] . These early genes encode transcription factors and activate transcription of late genes to establish tissue-specific outcomes [44] . While BR-C, E74 and E93 are required for salivary gland PCD, E93 functions as a stage-specific regulator of cell death and BR-C and E74 have wider developmental roles [25] , [44] , [45] , [46] . In particular, the transcription of rpr and dronc requires ecdysone-regulated early genes BR-C and E93 and not E74 (ref. 24 ). Given this we examined the expression of BR-C and E93 in dUTX 1 salivary glands. The levels of E93 were significantly decreased in dUTX 1 salivary glands at 14 h RPF while there was no significant change in the BR-C transcript levels compared with control ( Fig. 6a ). Furthermore, ChIP analysis revealed that dUTX was recruited to the E93 promoter and dUTX knockdown resulted in increased H3K27me3 ( Fig. 6b ). This suggests that dUTX plays a distinct role in both the early and the late transcriptional response to ecdysone. 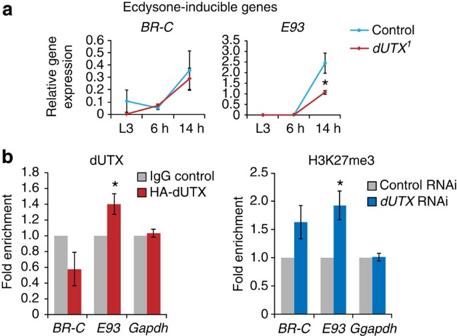Figure 6: dUTX regulates ecdysone-induced gene E93. (a) Levels ofBR-CandE93transcripts were measured in salivary glands isolated from third instar larvae (L3), 6 h and 14 h RPF control (blue line) anddUTX1(red line) using qPCR and expressed relative to the internal control generp49. (b) The occupancy of dUTX on the promoter regions ofBR-CandE93genes detected by ChIP. SL2 cells overexpressing HA-dUTX were chromatin-immunoprecipitated with anti-HA and anti-GFP (IgG control) antibodies following ecdysone treatment. Results are shown as the fold enrichment of % input compared with IgG control. In the right hand panel abundance of H3K27me3 on the promoters ofBR-CandE93genes as detected by ChIP is shown. SL2 cells knockdown fordUTX(dUTXRNAi) were chromatin-immunoprecipitated with anti-H3K27me3 and rabbit IgG (control) antibodies following ecdysone treatment. Results are shown as the fold enrichment of % input compared with RNAi control. Data in all panels are expressed as means from three independent experiments, with error bars representing s.e.m. *P<0.05 (Studentst-test). Figure 6: dUTX regulates ecdysone-induced gene E93. ( a ) Levels of BR-C and E93 transcripts were measured in salivary glands isolated from third instar larvae (L3), 6 h and 14 h RPF control (blue line) and dUTX 1 (red line) using qPCR and expressed relative to the internal control gene rp49 . ( b ) The occupancy of dUTX on the promoter regions of BR-C and E93 genes detected by ChIP. SL2 cells overexpressing HA-dUTX were chromatin-immunoprecipitated with anti-HA and anti-GFP (IgG control) antibodies following ecdysone treatment. Results are shown as the fold enrichment of % input compared with IgG control. In the right hand panel abundance of H3K27me3 on the promoters of BR-C and E93 genes as detected by ChIP is shown. SL2 cells knockdown for dUTX ( dUTX RNAi) were chromatin-immunoprecipitated with anti-H3K27me3 and rabbit IgG (control) antibodies following ecdysone treatment. Results are shown as the fold enrichment of % input compared with RNAi control. Data in all panels are expressed as means from three independent experiments, with error bars representing s.e.m. * P <0.05 (Students t -test). Full size image Demethylase activity of dUTX is required for cell death Consistent with the H3K27me3 demethylase activity of dUTX the level of H3K27me3 was increased in dUTX 1 . Mosaic clonal analysis revealed increased H3K27me3 immunostaining in dUTX 1 clones compared with the neighbouring wild-type cells ( Fig. 7a ), with only a small decrease in H3K4me1 ( Supplementary Fig. S5 ). The total levels of H3K27me3 were similarly increased in whole dUTX mutant salivary glands compared with the control ( Fig. 7b ). To determine whether the demethylase function of dUTX was required for salivary gland PCD, we expressed wild-type or JmjC domain mutant dUTX specifically in the salivary gland in a dUTX 1 background. The dUTX mutant JmjC domain (JmjC*) lacks two residues (His883 and Glu885) critical for its catalytic function [23] . While expression of the wild-type dUTX partially rescued the delayed salivary gland degradation of the dUTX mutant, the expression of the catalytically inactive dUTX did not ( Fig. 7c ). These findings support the role of dUTX catalytic activity in regulation of salivary gland PCD. 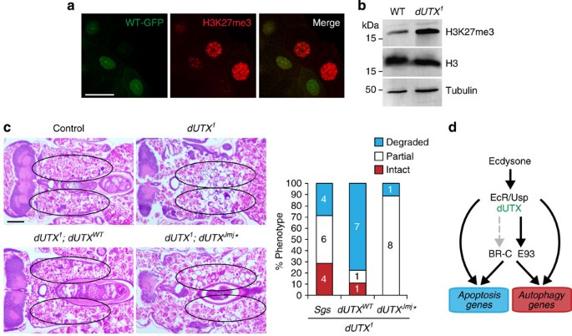Figure 7: dUTX demethylase activity is required for cell death. (a) Mosaic clones ofdUTX1(hsFLP; ubi-GFP FRT40A/dUTX1FRT40A)from third instar larval salivary glands with wild-type cells marked by nuclear-localized GFP (green).dUTX1clones have high levels of H3K27me3 (red) compared with the neighbouring control cells marked by GFP. Scale bar represents 50 μm. (b) Western blot analysis of the level of H3K27me3 in control anddUTX1larval salivary glands. Alpha-tubulin and H3 serve as loading controls. (c) Expression of dUTX wild-type (dUTXWT) and dUTX catalytic mutant (dUTXJmj) in the salivary glands (usingSgs3-GAL4driver) ofdUTX1. Histological analysis of paraffin sections at 24 h RPF shows intact salivary glands present indUTX1and indUTX1;dUTXJmj*compared with control anddUTX1;dUTXWTat 24 h RPF. Ovals indicate the position of salivary glands and fragments. Scale bar represent 50 μm. Quantification of the salivary gland phenotypic data at 24 h RPF is shown on the right. (d) A schematic representation of the role of dUTX in ecdysone-mediated transcriptional regulation of cell death genes, directly or via E93. Figure 7: dUTX demethylase activity is required for cell death. ( a ) Mosaic clones of dUTX 1 (hsFLP; ubi-GFP FRT40A/dUTX 1 FRT40A) from third instar larval salivary glands with wild-type cells marked by nuclear-localized GFP (green). dUTX 1 clones have high levels of H3K27me3 (red) compared with the neighbouring control cells marked by GFP. Scale bar represents 50 μm. ( b ) Western blot analysis of the level of H3K27me3 in control and dUTX 1 larval salivary glands. Alpha-tubulin and H3 serve as loading controls. ( c ) Expression of dUTX wild-type ( dUTX WT ) and dUTX catalytic mutant ( dUTX Jmj ) in the salivary glands (using Sgs3-GAL4 driver) of dUTX 1 . Histological analysis of paraffin sections at 24 h RPF shows intact salivary glands present in dUTX 1 and in dUTX 1 ; dUTX Jmj* compared with control and dUTX 1 ; dUTX WT at 24 h RPF. Ovals indicate the position of salivary glands and fragments. Scale bar represent 50 μm. Quantification of the salivary gland phenotypic data at 24 h RPF is shown on the right. ( d ) A schematic representation of the role of dUTX in ecdysone-mediated transcriptional regulation of cell death genes, directly or via E93. Full size image UTX function is known to be critical in mammalian embryonic development and somatic and germ cell reprogramming. Here we found a novel role for dUTX in steroid hormone-mediated cell death during development. Our study provides the novel observation that dUTX, together with nuclear hormone receptor EcR/Usp, is capable of regulating gene expression both spatially and temporally in a hormone-dependent manner. UTX gene mutations are frequently observed in malignancies including lethal castration-resistant prostate cancer [18] , [47] , although a role for UTX in androgen receptor-mediated transcription has not yet been identified [8] . Our study indicates that UTX is a good candidate to extend the investigation to examine the role of UTX in coordinating nuclear hormone receptor-regulated gene expression, particularly in androgen receptor-mediated transcription during mammalian development and hormone-dependent cancers. The complete degradation of larval salivary glands during metamorphosis utilizes both apoptosis and autophagy and by coordinately controlling the expression of critical genes in these two distinct biological pathways, dUTX ensures timely removal of salivary glands in response to temporal ecdysone pulse. The majority of studies addressing induction of autophagy have focused upon autophagosome formation and protein degradation. The transcriptional regulation of autophagy induction remains poorly understood. Indeed, several Atg genes are transcriptionally upregulated following autophagy induction; however, the molecular pathways are only beginning to be revealed. For example, the master gene controlling lysosomal biogenesis, transcription factor EB, coordinates the expression of both autophagy and lysosomal genes to induce autophagy in response to starvation [48] . More recently, induction of autophagy has been linked to reduced histone H4 lysine 16 acetylation (H4K16ac) through downregulation of the histone acetyltransferase hMOF [49] . Downregulation of H4K16 deacetylation was associated with the downregulation of several Atg genes, whereas antagonizing H4K16ac downregulation upon autophagy induction resulted in cell death. The study indicates that a specific histone modification during autophagy modulates the expression of Atg genes, and is important for survival versus death responses upon autophagy induction [49] . Our work now describes dUTX as another regulator of autophagy and cell death in the context of developmental PCD and in concert with the steroid hormone response. Future studies to understand the complex nuclear events regulating both repression and induction of autophagy gene expression in response to particular signals will be important. Despite the opposing roles of H3K27 and H3K4 methylation in transcriptional regulation, UTX has been identified in association with H3K4 methyltransferase and to play demethylase-independent functions [23] , [18] , [19] . Our study suggests that the demethylase activity of dUTX is necessary for hormone-mediated cell death. The nuclear hormone receptor response to ecdysone initiates a hierarchical transcription cascade by induction of transcription factors, including BR-C, E74 and E93. These transcription factors drive expression of downstream genes including cell death genes. Our data show that dUTX regulates E93 and suggests that this HDM can regulate cell death both directly, through the transcription of apoptosis and autophagy genes through direct recruitment via EcR/Usp, as well as indirectly through key transcription factor E93 ( Fig. 7d ). This additional level of regulation through the stage-specific transcription factor E93 may provide temporal control of ecdysone response during metamorphosis. The role of autophagy in cell death is a matter of considerable debate as autophagy is generally a cell survival mechanism in response to cellular stress and nutrient limitations [50] . Studies in Drosophila have provided perhaps some of the strongest evidence for a role of autophagy in developmental cell death in vivo . Our data presented in this paper demonstrating coordinate regulation of both key apoptosis and autophagy genes by a single histone-modifying enzyme further provide genetic and molecular evidence linking autophagy and apoptosis in PCD during metamorphosis. Cell culture and RNA interference SL2 cells were cultured in Schneider’s medium (GIBCO, Life Technologies, Carlsbad, CA, USA) supplemented with 10% FBS and 1% penicillin–streptomycin at 28 °C. Ecdysone (Sigma-Aldrich, St Louis, MO, USA) was used at 10 μM. For dsRNAi template 1 the region 1–531 bp and for dsRNAi template 2 the region 2,935–3,405 bp of dUTX-RA was cloned into pGEM-T (Promega, Madison, WI, USA) and double-stranded RNAs (dsRNA) were generated by in vitro transcription kit MEGAscript (Ambion, Life Technologies, Carlsbad, CA, USA) using T7/Sp6 polymerase. Control dsRNAi construct containing GFP in pGEM-T was as described [51] . For RNAi treatment, SL2 cells were washed once and resuspended in serum-free medium at 2 × 10 6 cells per ml. dsRNA (25 μg) was added to 1 ml of cell suspension and incubated for 3 h at 28 °C. After the incubation, 2 ml complete medium was added to the cells and cultured for another 48 h before harvesting the cells for RNA extraction or caspase assays. For cell viability SL2 cell suspension (20 μl) in Schneider media was incubated with equal volume of trypan blue and counted on haemocytometer or with 180 μl of Muse Count & Viability Reagent for 5 min at room temperature and analysed using Muse (Millipore, Billerica, MA, USA) instrument. For expression of HA-tagged dUTX in SL2 cells, dUTX was cloned into the Drosophila Gateway vector collection pAWH (containing Actin5C promoter with C-terminal 3 × HA epitopes) according to the Gateway Technology manual (Invitrogen, Life Technologies, Carlsbad, CA, USA). Briefly, dUTX was amplified using dUTX -F 5′-CACCATGGGGCAACTAACTTTCGAAG-3′ and dUTX -R 5′-CTGAGTGTATGCTAGTCGTTGG-3′ primers and cloned into pENTR/SD/D-TOPO (Invitrogen). The resulting entry clone, pENTR-dUTX, was then recombined with pAWH destination vector using Gateway LR Clonase Enzyme Mix (Invitrogen). Quantitative real-time PCR Quantification of gene expression and the level of RNAi knockdown of various lines was performed by qPCR. Total RNA was isolated from Drosophila salivary glands and SL2 cells using TRIzol reagent (Invitrogen). cDNA was synthesized using High Capacity cDNA Reverse Transcription Kit (Applied Biosciences, Life Technologies) and oligo dT primer (Geneworks, Thebarton, SA, Australia), with 1 μg of total RNA. Briefly, qPCR was performed using 2 μl of cDNA and 5 μl of RT [2] Real-Time SYBR Green/ROX PCR MasterMix (Qiagen, Valencia, CA, USA) in 10 μl reactions on a Rotor-Gene 6000 (Corbett Research, Mortlake, NSW, Australia). Reactions were performed in triplicate and the mRNA expression levels were normalized against the internal control gene rp49 using the ΔΔCT method. Primer sets used are described in Supplementary Table S1 . Caspase activity assays The caspase activity assays were performed as previously described [52] , using 70 μg of salivary gland protein lysate or 50 μg of total protein lysate from SL2 cells with 100 μM of DEVD-AMC (MP Biomedicals, Solon, OH, USA) made up to a final volume of 100 μl in caspase assay buffer (50 mM HEPES, pH 7.5, 100 mM NaCl, 1 mM EDTA, 0.1% CHAPS, 10% sucrose, 5 mM DTT, 0.5% TritonX-100, 4% glycerol with protease inhibitor mix (Roche, Indianapolis, IN, USA)). The fluorescence was measured at 30 min intervals over a 3 h time course using a FluoStar spectrophotometer (BD Biosciences, Franklin Lakes, NJ, USA) (excitation, 385 nm; emission, 460 nm). The change in DEVD-AMC fluorescence over time was plotted to determine the linear slope of the line that was multiplied by the conversion factor and the reaction volume expressed as pmol substrate per min (ref. 52 ). The conversion factor was calculated as the inverse of the slope of the standard curve obtained by plotting the fluorescence reading of the serial dilutions (5, 10, 25, 50 and 100 μM) of DEVD-AMC [52] . GST pull-down For the expression of recombinant dUTX–NR region as GST fusion protein, the sequence corresponding to amino acids 820–1,136 was cloned into pGEX-2T using primers for dUTX–NR 5′-AGGCAAGGATCCAGGTTCGGGACCAACGTGGACCTCTCC-3′ and 5′-AGGCAAGGATCCCTGAGTGTATGCTAGTCCTTGGG-3′. To generate 35 S-labelled EcR and Usp, the pCMX-EcR [53] and pCMX-Usp [53] templates were used with the TNT Coupled Reticulocyte Lysate System (Promega) in the presence of 35 S-Methionine (MP Biomedicals). Chromatin immunoprecipitation For chromatin immunoprecipitation (ChIP), ~6 × 10 6 SL2 cells were fixed in 1% formaldehyde at room temperature for 10 min, then glycine was added to a final concentration of 0.125 M and incubated for a further 5 min. Cells were washed thrice in ice-cold PBS and lysed in cell lysis buffer (1% SDS, 10 mM EDTA, 50 mM Tris–HCl (pH 8.1) and complete protease inhibitors cocktails (Roche)). The cell lysate was sonicated for 25 min (30 s on/off) using Bioruptor (Diagenode, Liège, Belgium) to shear the chromatin into 200–500 bp fragments. The chromatin solution was then clarified and pre-cleared by incubating with protein G agarose beads for 1 h at 4 °C. Two micrograms of antibodies anti-HA, anti-EcR-B1 (AD4.4, Developmental Studies Hybridoma Bank, Iowa, IA, USA), anti-H3K27me3 (Abcam, Cambridge, UK) and anti-GFP (Roche) were used for each ChIP reaction and incubated overnight at 4 °C. The protein G beads were prepared by incubating with BSA and salmon sperm DNA before adding into the ChIP reactions and incubated for 2 h at 4 °C. The beads were washed once in low-salt wash buffer (0.1% SDS, 1% Triton X-100, 2 mM EDTA, 20 mM Tris-HCl (pH 8.1), 150 mM NaCl), high-salt wash buffer (0.1% SDS, 1% Triton X-100, 2 mM EDTA, 20 mM Tris–HCl (pH 8.1), 500 mM NaCl), LiCl wash buffer (250 mM LiCl, 1% NP40, 1% deoxycholate, 1 mM EDTA, 10 mM Tris–HCl (pH 8.1)) and twice in TE buffer (10 mM Tris-HCl, 1 mM EDTA (pH 8.0)). The immunoprecipitated DNA was eluted from the beads in freshly prepared elution buffer (0.1 M NaHCO 3 and 1% SDS). The eluates were then reverse-crosslinked by incubating at 65 °C overnight. The DNA was purified by phenol–chloroform extraction and ethanol precipitation. The precipitated DNA was then analysed by qPCR and the promoter recruitment is expressed as the fold enrichment over control IgG normalized by the input DNA. Primer sequences for qPCR are listed in Supplementary Table S2 . Co-immunoprecipitation Cells transfected with pAWH-dUTX-HA were lysed in cell lysis buffer (20 mM Tris–HCl (pH 7.8), 100 mM NaCl, 0.5% NP40, 5% glycerol, 1 mM EDTA and complete protease inhibitors cocktails from Roche) for 15 min on ice. The nuclear fraction was pelleted by centrifugation at 13,000 r.p.m. for 30 s at 4 °C and lysed in nuclear lysis buffer (20 mM Tris–HCl (pH 7.4), 400 mM NaCl, 7.5 mM MgCl 2 , 0.2 mM EDTA, 0.1 mM EGTA, 1 mM DTT with complete protease inhibitors cocktail (Roche)) for 45 min at 4 °C. Both cytoplasmic and nuclear lysates were combined and 1 mg of total proteins was immunoprecipitated with 10 μg anti-HA antibodies (Roche, cat. no. 11583816001) or anti-Myc antibodies (Roche, cat. no. 1166720300) as a control, overnight at 4 °C. The protein G agarose beads were added to the reaction and the immune complexes were precipitated by incubating for 1 h at room temperature. The agarose beads were washed once in PBS supplemented with 1 mM CaCl 2 and 1 mM MgCl 2 , and then boiled in 2 × SDS loading buffer before immunoblotting. Immunoblotting Total protein (50–100 μg) in SDS protein buffer (100 mM Tris–HCl (pH 6.8), 200 mM dithiothreitol, 4% SDS, 0.2% bromophenol blue, 20% glycerol) was resolved by SDS–PAGE and transferred to polyvinylidine difluoride membrane. Membranes were blocked in 5% skim milk-TBST (tris-buffered saline in 0.05% Tween20) and incubated with a 1 in 1,000 dilution of the following primary antibodies: rabbit anti-H3 (Cell Signalling Technology, Danvers, MA, USA), rabbit anti-H3K27me3 (Millipore), mouse anti-EcR-B1 (AD4.4, Developmental Studies Hybridoma Bank) and anti-α tubulin (Abcam). Secondary antibodies were anti-rabbit AP (Millipore) and anti-mouse AP (Millipore) used at 1 in 2000 dilution. Proteins were detected by enhanced chemifluorescence or enhanced chemiluminescence (ECL-Plus, Amersham/Pharmacia, Piscataway, NJ, USA). Original immunoblots are shown in Supplementary Figure S6 . Fly stocks dUTX 1 , dUTX 2 and UAS-dUTX , UAS-dUTX jmjC are described [16] . The following stocks were from the Bloomington stock centre (Bloomington, IN, USA): w 1118 , hsFLP; ubi-GFP FRT40A , Sgs3-GAL4 , UAS-EcR-RNAi 104. All flies were maintained and crosses performed at 25 °C. Measurement of ecdysone titre Pupae (six pupae per set) were collected for both control and dUTX 1 mutant at 12 h RPF, snap-frozen in liquid nitrogen and stored at −80 °C. The pupae were weighed before extracting ecdysteroid. Samples were homogenized in 300 μl of methanol and centrifuged at 16,000 g for 20 min at 4 °C. This was repeated twice and the combined methanol supernatants were dried before resuspending in enzyme immunoassay (EIA) buffer (Cayman Chemicals, Inc., USA). Ecdysteroid levels were measured as 20E (Sigma-Aldrich, USA) equivalents. The assay was performed using 20-hydroxyecdysone antiserum, 20-hydroxyecdysone AChE Tracer and Ellmann reagent (all from Cayman Chemicals, Inc., USA). Briefly, 50 μl of the standards and diluted samples were incubated with 50 μl of tracer and anti-serum in anti-rabbit IgG coated ELISA plates overnight, washed five times and developed by adding 200 μl Ellman’s reagent. The absorbance was read at 405 nm and all assays were performed in triplicate. Histology For hematoxylin and eosin staining of whole pupal sections, 14 h and 24 h RPF pupae were fixed in FAAG (85% ethanol, 4% formaldehyde, 5% acetic acid and 1% glutaraldehyde), then paraffin-embedded prior to sectioning and then hematoxylin and eosin-stained [27] . The controls were w 1118 Drosophila alone and crossed to Sgs3-GAL4 . For each genotype a minimum of 10 pupae were examined using a stereozoom microscope (Olympus, Tokyo, Japan). Immunohistochemistry Salivary glands of the required genotype were dissected from appropriately staged animals in PBS then fixed with 4% paraformaldehyde in PBS for 20 min at room temperature. Primary antibodies were rabbit anti-cleaved caspase-3 (Cell signalling, #9661), rabbit anti-H3K27me3 (Millipore) and anti-Lamin Dm0 (DSHB, ADL67.10) used at 1 in 100 dilution. Secondary antibodies were anti-rabbit Alexa-FLUOR 488, anti-rabbit Alexa-FLUOR 568 and anti-mouse Alexa-FLUOR 568 (Molecular Probes, Eugene, CA, USA) used at 1 in 200 dilution. Hoechst 33342 (Sigma-Aldrich) was used to stain DNA. The samples were imaged with a Biorad confocal microscope (Bio-Rad Microscience, UK; at Detmold Imaging Core Facility, Hanson Institute, Adelaide, SA, Australia). Polytene chromosome immunostaining Salivary glands from third instar larvae were dissected and fixed on coverslips in 4% paraformaldehyde in 45% glacial acetic acid for 5–10 min. The coverslips were placed on a microscope slide and then the chromosomes were spread using a blunt pair of forceps. The slides were then submerged in liquid nitrogen before removing the coverslip. The samples were blocked in 0.5% Bovine Serum Albumin 0.1% Triton-X in PBS (PBT) for 1 h prior to incubation with 1 in 100 dilution of anti-EcR-B1 and anti-dUTX [23] overnight at 4 °C. Secondary antibodies were anti-rabbit Alexa-FLUOR 488, and anti-mouse Alexa-FLUOR 568 (Molecular Probes, Eugene, CA, USA) used at 1 in 200 dilution. Hoechst 33342 (Sigma-Aldrich) was used to stain DNA. The samples were imaged by confocal microscopy (Detmold Imaging Core Facility, Hanson Institute, Adelaide, SA, Australia). Live mCherry imaging To assay for mCherry-Atg8a, salivary glands were dissected in PBS with Hoechst 33342 (Sigma-Aldrich) to stain DNA and imaged immediately. Images were quantificated using the mean value from histogram function in Photoshop per cell, which represents the average intensity value. Imaging Confocal images were obtained using a BioRad Radiance 2100 confocal microscope with Argon ion 488 nm (14 mw) and Green HeNe 543 nm (1.5 mw) lasers and an Olympus IX70 inverted microscope with a × 40 UPLAPO (NA=1.2 water) objective. The dual labelled samples were imaged with two separate channels (PMT tubes) in a sequential setting. Green fluorescence was excited with an Ar 488 nm laser line and the emission viewed through a HQ515/30 nm narrow band barrier filter in PMT1. Red fluorescence was excited with a HeNe 543 nm laser line and the emission viewed through a long-pass barrier filter (E570LP) in PMT2. Automatically all signals from PMTs 1 and 2 were merged. Images were captured using Confocal Assistant software for Microsoft Windows (Todd Clark Brelje, Bethesda, MD, USA) and compiled using Photoshop CS5 (Adobe). Statistical analysis of data Student’s t -test, two-tailed equal variance, was used for all statistical analysis unless otherwise stated. Data are expressed as mean±s.d. or mean±s.e.m., as appropriate. P <0.05 was considered significant. χ 2 analysis was performed using an online calculation chi-square tool. How to cite this article: Denton, D. et al. UTX coordinates steroid hormone-mediated autophagy and cell death. Nat. Commun. 4:2916 doi: 10.1038/ncomms3916 (2013).